LIS1-dependent retrograde translocation of excitatory synapses in developing interneuron dendrites Synaptic remodelling coordinated with dendritic growth is essential for proper development of neural connections. After establishment of synaptic contacts, synaptic junctions are thought to become stationary and provide fixed anchoring points for further dendritic growth. However, the possibility of active translocation of synapses along dendritic protrusions, to guide the proper arrangement of synaptic distribution, has not yet been fully investigated. Here we show that immature dendrites of γ-aminobutyric acid-positive interneurons form long protrusions and that these protrusions serve as conduits for retrograde translocation of synaptic contacts to the parental dendrites. This translocation process is dependent on microtubules and the activity of LIS1, an essential regulator of dynein-mediated motility. Suppression of this retrograde translocation results in disorganized synaptic patterns on interneuron dendrites. Taken together, these findings suggest the existence of an active microtubule-dependent mechanism for synaptic translocation that helps in the establishment of proper synaptic distribution on dendrites. The establishment of neural networks depends on the formation, elimination and remodelling of synapses [1] , [2] . In mature pyramidal neurons, most excitatory synapses are located on the heads of dendritic spines [3] . During development, immature dendrites of pyramidal neurons are first covered with motile filopodia [4] , [5] . Because filopodia can make initial contact with axons [5] , [6] and their expression precedes that of spines [7] , it has been proposed that filopodia may function as spine precursors. Imaging studies have captured the retraction of some filopodia into spine-like protrusions and this may reflect direct transition of filopodia into spines [5] , [8] . However, electron microscopic analysis of in vivo synapse formation supported a role for filopodia in the formation of shaft synapses, which subsequently develop into mature spine synapses [7] . These studies indicate that filopodia may be important during the initial search for appropriate axons, but the development of mature spine synapses may require dynamic morphological changes of both dendrites and nascent synapses [9] . Although development of spine synapses is considered the canonical model of glutamatergic synapse formation, many neuronal types in the vertebrate CNS receive glutamatergic innervation directly on the dendritic shafts. Among this population are non-pyramidal GABAergic (γ-aminobutyric acid) interneurons that account for 10–25% of all neurons in the mammalian neocortex and hippocampus [10] , [11] , and have a crucial role in information processing through local suppression of pyramidal neuronal activity. Most subtypes of GABAergic interneurons have few if any spines, although their dendritic shafts are densely covered with glutamatergic synapses. In fact, the density of glutamatergic synapses on the dendrites of parvalbumin-positive fast-spiking interneurons has been estimated to be 3.4 per μm [12] , which exceeds the average density of excitatory inputs onto pyramidal neuron dendrites (2–3 per μm) [3] , [13] . How do interneurons acquire such a dense covering of glutamatergic synapses? One possible explanation is that immature interneurons generate dendritic filopodia that initiate axonal contact and then retract after establishing stable synaptic contacts. However, there is no experimental evidence supporting this model. Alternatively, shaft synapses may be generated directly, without the intermediate step of filopodial contact. GABAergic synaptic contacts on pyramidal neurons are generated directly on dendritic shafts [14] . The complex and tortuous trajectories of GABAergic axons may facilitate frequent direct contact with the dendritic shafts of pyramidal neurons. On the other hand, glutamatergic axons take more linear trajectories, which may necessitate additional mechanisms within interneuron dendrites to increase the likelihood of making contact with glutamatergic axons. To explore the mechanisms of glutamatergic synapse formation on interneuron dendrites, time-lapse imaging of postsynaptic densities (PSDs) and dendritic protrusions was performed. Interneuron dendrites formed long-lasting protrusions that guided retrograde translocation of synaptic contacts to the parental dendrites. Pharmacological and genetic analyses revealed that the translocation process was dependent on microtubules and the activity of LIS1, an essential regulator of dynein-mediated mobility [15] , [16] . These findings suggest that interneurons use both active dendritic protrusions and microtubule-dependent synaptic mobility to establish the proper distribution of glutamatergic inputs. PSD-containing dendritic protrusions in immature interneurons To analyse dendritic morphology and PSD distribution in developing interneurons, we investigated two independent culture systems, dissociated cultures of embryonic mouse hippocampal neurons and organotypic slice cultures of the newborn mouse neocortex. It is important to reliably discriminate inhibitory interneurons from excitatory neurons in both culture systems. In dissociated cultures, the transmitter phenotype of putative interneurons was evaluated by immunocytochemical staining of the 67-kDa isozyme of glutamate decarboxylase GAD67 ( Fig. 1a ). In cortical slices, immunocytochemistry with GAD67 was not feasible because of the limited penetration of antibodies. Therefore, we transfected red fluorescent protein (RFP) into cortical slices from GAD67-GFP knockin mice ( Fig. 1a ) and transfected neurons were classified as pyramidal or non-pyramidal based on morphology, whereas their transmitter phenotype was determined by green fluorescent protein (GFP). We found that 87% (39/45) non-pyramidal neurons expressed GFP, whereas only 3% (5/176) pyramidal-shaped neurons expressed GFP (total neurons examined from eight cortical slices). Thus, morphological classification was a reliable method for identification of GABAergic interneurons. 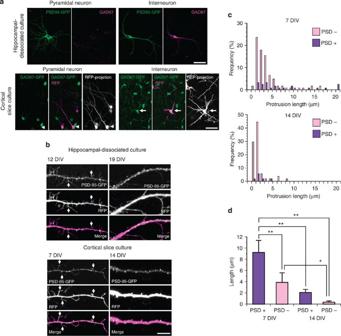Figure 1: Developmental change in dendritic morphology and PSD distribution in interneurons. (a) Upper right panel: a hippocampal-dissociated neuron expressing PSD-95-GFP with the typical morphology of an interneuron. The GABAergic phenotype of this neuron was confirmed by anti-GAD67 immunostaining. Upper left panel: a GAD67-negative neuron extending branched dendrites in a dissociated culture. This neuron exhibits the typical morphology of hippocampal pyramidal neurons in culture. Lower right panel: RFP expression in layer II–III non-pyramidal neurons in cortical slices prepared from GAD67-GFP knockin mice. The RFP-positive non-pyramidal neuron (arrows) was also GFP-positive, indicating its GABAergic transmitter phenotype. Lower left panel: RFP-expressing pyramidal-shaped neuron (arrowheads) was GFP-negative. Scale bars, 50 μm. (b) Distribution of PSD-95-GFP puncta and dendritic protrusions in non-pyramidal neurons in a dissociated hippocampal culture at 12 and 19 DIV and a cortical slice culture at 7 and 14 DIV. Dendritic protrusions (arrows) were specifically enriched in immature dendrites and were positive for PSD-95-GFP puncta. Scale bar, 10 μm. (c) Distribution of protrusion lengths in cortical slices at 7 and 14 DIV. At both time points, 2–4 dendritic segments of 12 neurons from 4 slices were imaged and the same number of dendritic protrusions was randomly selected for quantification. (d) The mean lengths of dendritic protrusions at 7 and 14 DIV with or without PSD-95-GFP puncta (PSD+ or PSD−;n=12 neurons from 4 slices at both time points). Significant differences (one-way analysis of variance followed by Tukey–Kramer multiple comparison tests): *P<0.05; **P<0.01. All numeric data are mean±s.e.m. Figure 1: Developmental change in dendritic morphology and PSD distribution in interneurons. ( a ) Upper right panel: a hippocampal-dissociated neuron expressing PSD-95-GFP with the typical morphology of an interneuron. The GABAergic phenotype of this neuron was confirmed by anti-GAD67 immunostaining. Upper left panel: a GAD67-negative neuron extending branched dendrites in a dissociated culture. This neuron exhibits the typical morphology of hippocampal pyramidal neurons in culture. Lower right panel: RFP expression in layer II–III non-pyramidal neurons in cortical slices prepared from GAD67-GFP knockin mice. The RFP-positive non-pyramidal neuron (arrows) was also GFP-positive, indicating its GABAergic transmitter phenotype. Lower left panel: RFP-expressing pyramidal-shaped neuron (arrowheads) was GFP-negative. Scale bars, 50 μm. ( b ) Distribution of PSD-95-GFP puncta and dendritic protrusions in non-pyramidal neurons in a dissociated hippocampal culture at 12 and 19 DIV and a cortical slice culture at 7 and 14 DIV. Dendritic protrusions (arrows) were specifically enriched in immature dendrites and were positive for PSD-95-GFP puncta. Scale bar, 10 μm. ( c ) Distribution of protrusion lengths in cortical slices at 7 and 14 DIV. At both time points, 2–4 dendritic segments of 12 neurons from 4 slices were imaged and the same number of dendritic protrusions was randomly selected for quantification. ( d ) The mean lengths of dendritic protrusions at 7 and 14 DIV with or without PSD-95-GFP puncta (PSD+ or PSD−; n =12 neurons from 4 slices at both time points). Significant differences (one-way analysis of variance followed by Tukey–Kramer multiple comparison tests): * P <0.05; ** P <0.01. All numeric data are mean±s.e.m. Full size image To investigate developmental changes in dendritic morphology and PSD distribution, dissociated hippocampal neurons at 12 and 19 days in vitro (DIV) and cortical slices at 7 and 14 DIV were analysed by fluorescence microscopy. We transfected neurons with GFP-tagged PSD-95, a marker of PSD, together with RFP as a volume label for morphological identification. As reported previously, mature interneurons maintained for more than 2 weeks in culture possessed few dendritic protrusions, and PSD-95 clusters were localized on dendritic shafts ( Fig. 1b ). Surprisingly, the morphology of immature interneuron dendrites was distinct; they expressed numerous filopodia-like protrusions from various positions along the dendritic shafts ( Fig. 1b ). These protrusions frequently contained PSD-95-GFP puncta. This transitional dendritic morphology and PSD distribution pattern was observed in both dissociated hippocampal interneurons and interneurons within cortical slices. Thus, transient formation of PSD-containing filopodia-like protrusions is likely to be a characteristic feature of forebrain GABAergic interneurons. To examine developmental changes in these filopodia-like protrusions, dendritic morphology and PSD distribution were quantitatively evaluated in cortical slices at 7 and 14 DIV. At 7 DIV, 24% dendritic protrusions of immature interneurons were longer than 5 μm ( Fig. 1c , 7 DIV). This fraction increased to 50% when we excluded protrusions without PSD-95-GFP puncta. Calculation of the average length confirmed the difference between protrusions with or without PSD-95-GFP puncta ( Fig. 1d ). The fraction of protrusions longer than 5 μm decreased from 24% at 7 DIV to only 5% at 14 DIV ( Fig. 1c , 14 DIV). The average protrusion length also decreased significantly during this developmental period, irrespective of the presence of PSD-95-GFP puncta ( Fig. 1d ). Thus, there is a developmental change in the morphology of dendritic protrusions. Dendritic protrusions appeared to occur less frequently later in development. The density of dendritic protrusions decreased significantly from 0.16±0.023 per μm at 7 DIV to 0.054±0.006 per μm at 14 DIV ( P <0.01, n =12 cells). Conversely, the density of PSD-95-GFP clusters increased significantly during the same developmental period from 0.23±0.035 per μm to 0.40±0.047 per μm ( P <0.01, n =12 cells). This result is consistent with the idea that long PSD-containing protrusions in immature interneurons have a special role in increase of shaft PSDs. Dynamics of dendritic protrusions in immature interneurons To reveal dynamic properties of interneuron dendritic protrusions, we recorded time-lapse images of immature interneurons expressing RFP in both dissociated cultures from wild-type embryos or cortical slices from GAD67-GFP knockin mice ( Fig. 2a,b , Supplementary Videos 1 and 2 ). Dendritic protrusions from interneurons exhibited dynamic morphological changes similar to the filopodia observed on pyramidal neuron dendrites. Both forms of protrusions were highly motile, generally <10 μm in length, and either unbranched or possessing a few side branches. Cumulative histograms of protrusion lengths and lifetimes ( Fig. 2c,d ) indicate that longer and stable protrusions were more frequent in interneurons. Interneuron protrusions were longer than those measured on pyramidal neurons (4.8±0.27 versus 3.8±0.20 μm, n =15 cells each, P <0.05) and the mean lifetime was higher (18.6±1.5 versus 11.6±1.2 min, n =15 cells each, P <0.01). However, two-dimensional plots of protrusion lengths and lifetimes revealed extensive overlap between these two types of neuron ( Fig. 2e,f ), suggesting that the differences in average protrusion length and lifetimes do not reflect the existence of distinct classes of protrusions. 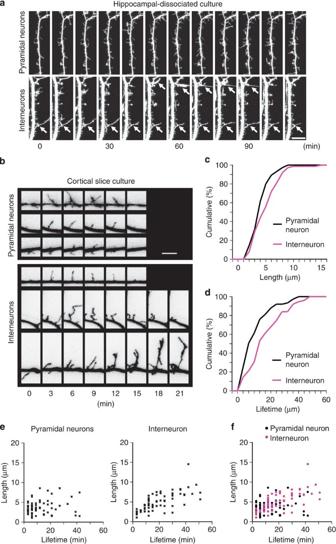Figure 2: Dynamics of dendritic protrusions in pyramidal neurons and interneurons. (a) Time-lapse images of protrusions in pyramidal neurons and interneurons expressing RFP at 9–12 DIV in dissociated cultures. Confocal image stacks were obtained every 10 min, and maximum-intensity projection images were generated. Arrows indicate typical dendritic protrusions on interneurons. Scale bar, 10 μm. (b) Time-lapse images of protrusive activity in pyramidal neurons and interneurons expressing RFP at 6–9 DIV in slices. Before image acquisition, the identities of the neurons were confirmed by GAD67-GFP fluorescence. Confocal image stacks were obtained every 3 min, and maximum-intensity projection images were generated. Scale bar, 5 μm. (c,d) Cumulative frequency plots of dendritic protrusion length and lifetime. Dendritic protrusions in interneurons were longer and more stable than those in pyramidal neurons. From the images of one to three dendritic segments of a single cell, five protrusions were randomly selected. For both interneurons and pyramidal neurons, data from 15 neurons were pooled and compared. (e) Two-dimensional plots of protrusion lifetime and length. Stable interneuron protrusions tend to be longer. (f) Overlay of two-dimensional plots of protrusion lifetime and length. The extensive overlap of data points suggests that the differences in average lengths and lifetimes do not reflect the existence of distinct classes of protrusions in interneurons. Figure 2: Dynamics of dendritic protrusions in pyramidal neurons and interneurons. ( a ) Time-lapse images of protrusions in pyramidal neurons and interneurons expressing RFP at 9–12 DIV in dissociated cultures. Confocal image stacks were obtained every 10 min, and maximum-intensity projection images were generated. Arrows indicate typical dendritic protrusions on interneurons. Scale bar, 10 μm. ( b ) Time-lapse images of protrusive activity in pyramidal neurons and interneurons expressing RFP at 6–9 DIV in slices. Before image acquisition, the identities of the neurons were confirmed by GAD67-GFP fluorescence. Confocal image stacks were obtained every 3 min, and maximum-intensity projection images were generated. Scale bar, 5 μm. ( c , d ) Cumulative frequency plots of dendritic protrusion length and lifetime. Dendritic protrusions in interneurons were longer and more stable than those in pyramidal neurons. From the images of one to three dendritic segments of a single cell, five protrusions were randomly selected. For both interneurons and pyramidal neurons, data from 15 neurons were pooled and compared. ( e ) Two-dimensional plots of protrusion lifetime and length. Stable interneuron protrusions tend to be longer. ( f ) Overlay of two-dimensional plots of protrusion lifetime and length. The extensive overlap of data points suggests that the differences in average lengths and lifetimes do not reflect the existence of distinct classes of protrusions in interneurons. Full size image Retrograde translocation of PSDs along dendritic protrusions Shaft synapses on mature interneuron dendrites may be formed by direct contact of growing axons with dendritic shafts or through the interaction of dendritic protrusions with surrounding axons and subsequent transfer of synapses to dendritic shafts. To discriminate between these two possible mechanisms, we monitored the behaviour of GFP-labelled PSD puncta in immature interneurons maintained in a dissociated culture from 9 to 12 DIV and in slices from 4 to 9 DIV. Time-lapse imaging of fluorescent PSD puncta labelled by either PSD-95-GFP or another GFP-tagged PSD scaffold protein, Homer1c, revealed retrograde translocation of these nascent postsynaptic molecular complexes along dendritic protrusions both in dissociated hippocampal cultures ( Fig. 3a ) and in cortical organotypic slice preparations ( Fig. 3b ). These moving PSD puncta occasionally reached the dendritic shafts ( Fig. 3a,b ). Local photoactivation of PSD-95 tagged with Dronpa indicated limited dissociation of PSD-95 from moving PSD. After transfer of PSD puncta to the parental dendritic shafts, the protrusions tended to become shorter and disappeared ( Supplementary Fig. S1 ). This observation suggests that the stability of protrusions and retrograde movement of PSDs are regulated by a common underlying mechanism. Although short-range anterograde displacement of puncta was occasionally observed, long-range translocation of PSD puncta was exclusively towards the base of protrusions ( Fig. 3c,d ). We recorded the relative positions of the PSD-95 puncta and classified puncta showing unidirectional movement >3 μm within 2 h towards the parental dendritic shafts as mobile puncta. The fraction of mobile PSD puncta was lower in mature dendrites ( Fig. 3e,f ). The velocity of PSD puncta was maintained, but mean translocation distance tended to be shorter in mature dendrites. Thus, immature interneuron dendrites possess a developmental stage-specific strategy for synaptogenesis entailing both the generation of long dendritic protrusions and the active retrograde translocation of postsynaptic structures towards the parental dendritic shafts. 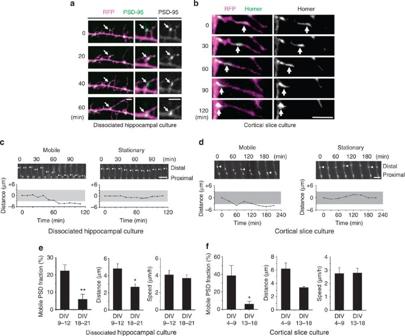Figure 3: PSD mobility in hippocampal-dissociated cultures and cortical slice cultures. (a) Time-lapse images of an interneuron dendrite expressing PSD-95-GFP and RFP in a dissociated hippocampal culture. A PSD-95-GFP punctum (arrows) moved in a distal to proximal direction towards the dendritic shaft. Scale bar, 3 μm. (b) Time-lapse images of an interneuron dendrite expressing GFP-Homer1c and RFP in a cortical slice culture. A GFP-Homer1c punctum (arrows) moved in a distal to proximal direction towards a stationary punctum at the base of a protrusion. Scale bar, 5 μm. (c,d) Distinct behaviours of mobile and stationary PSD-95-GFP puncta. Mobile PSD puncta showed unidirectional movement of >3 μm in distance (shaded area). Stationary PSD puncta showed limited lateral movement along dendritic protrusion with no preferred direction. Scale bars, 5 μm. (e) The mobile fraction and translocation distance of PSD-95 clusters, but not translocation speed, were lower in dissociated hippocampal interneurons at 18–21 DIV than at 9–12 DIV. (n=16 cells at 9–12 DIV,n=8 cells at 18–21 DIV. The number of PSD-95-positive protrusions/PSD-95 puncta analysed per cell was 2–8 protrusions/2–10 puncta at 9–12 DIV and 2–8 protrusions/3–12 puncta at 18–21 DIV.) Significant differences (unpaired Student'st-test): *P<0.05; **P<0.01. (f) The mobile fraction of PSD-95 clusters in cortical slice preparations was lower at 13–18 DIV than at 4–9 DIV. Translocation distance of PSD-95 clusters was lower in interneurons at 13–18 DIV compared with 4–9 DIV, but the difference was not statistically significant. The speed of translocation was comparable at both developmental stages. (n=16 cells from 16 slice cultures at DIV 4–9,n=5 cells from 5 slice cultures at DIV 13–18. The number of PSD-95-positive protrusions/PSD-95 puncta analysed per cell was 1–5 protrusions/2–9 puncta at DIV 4–9 and 3–8 protrusions/4–14 puncta at DIV 13–18.) Significant differences (unpaired Student'st-test): *P<0.05. All numeric data are mean±s.e.m. Figure 3: PSD mobility in hippocampal-dissociated cultures and cortical slice cultures. ( a ) Time-lapse images of an interneuron dendrite expressing PSD-95-GFP and RFP in a dissociated hippocampal culture. A PSD-95-GFP punctum (arrows) moved in a distal to proximal direction towards the dendritic shaft. Scale bar, 3 μm. ( b ) Time-lapse images of an interneuron dendrite expressing GFP-Homer1c and RFP in a cortical slice culture. A GFP-Homer1c punctum (arrows) moved in a distal to proximal direction towards a stationary punctum at the base of a protrusion. Scale bar, 5 μm. ( c , d ) Distinct behaviours of mobile and stationary PSD-95-GFP puncta. Mobile PSD puncta showed unidirectional movement of >3 μm in distance (shaded area). Stationary PSD puncta showed limited lateral movement along dendritic protrusion with no preferred direction. Scale bars, 5 μm. ( e ) The mobile fraction and translocation distance of PSD-95 clusters, but not translocation speed, were lower in dissociated hippocampal interneurons at 18–21 DIV than at 9–12 DIV. ( n =16 cells at 9–12 DIV, n =8 cells at 18–21 DIV. The number of PSD-95-positive protrusions/PSD-95 puncta analysed per cell was 2–8 protrusions/2–10 puncta at 9–12 DIV and 2–8 protrusions/3–12 puncta at 18–21 DIV.) Significant differences (unpaired Student's t -test): * P <0.05; ** P <0.01. ( f ) The mobile fraction of PSD-95 clusters in cortical slice preparations was lower at 13–18 DIV than at 4–9 DIV. Translocation distance of PSD-95 clusters was lower in interneurons at 13–18 DIV compared with 4–9 DIV, but the difference was not statistically significant. The speed of translocation was comparable at both developmental stages. ( n =16 cells from 16 slice cultures at DIV 4–9, n =5 cells from 5 slice cultures at DIV 13–18. The number of PSD-95-positive protrusions/PSD-95 puncta analysed per cell was 1–5 protrusions/2–9 puncta at DIV 4–9 and 3–8 protrusions/4–14 puncta at DIV 13–18.) Significant differences (unpaired Student's t -test): * P <0.05. All numeric data are mean±s.e.m. Full size image In dissociated cultures, 85–91% of PSD-95-GFP puncta were associated with presynaptic markers ( Supplementary Fig. S2 ). In cortical slices, 78–80% of PSD-95-GFP clusters in dendritic protrusions were also associated with presynaptic markers. Furthermore, a large fraction of PSD-95-positive protrusions (88–93%) were in contact with presynaptic markers (synapsin I, synaptophysin) in two types of cultures. These results indicate that the majority of imaged PSD puncta were already associated with presynaptic axons. To confirm the simultaneous movement of presynaptic and postsynaptic components, we also recorded time-lapse images of PSD-95-YFP puncta in postsynaptic neurons together with synaptophysin-CFP puncta in axons that are in contact ( Fig. 4a ). These two fluorescent probes were expressed in only a subset of neurons in dissociated culture by recombinant adenovirus-mediated transfection [6] ; therefore, only a fraction of synaptic junctions showed co-localization of these presynaptic and postsynaptic markers. The movement of PSD-95-YFP and synaptophysin-CFP puncta was highly coordinated ( Fig. 4b ). The fraction of mobile pairs of PSD-95-YFP puncta and synaptophysin-CPF puncta was comparable with the total mobile fraction of PSD-95-YFP puncta and that of synaptophysin-CFP puncta ( Fig. 4c ). This result excludes the possibility that PSD-95 clusters with synaptic contacts were less motile in comparison with clusters without contacts. To confirm the presence of functional presynaptic structures, we labelled active presynaptic sites by FM1-43. The movement of PSD-95-TagRFP was highly correlated with that of FM1-43 puncta ( Fig. 4d and e ), and the average velocity of FM1-43 puncta was comparable to that of PSD-95-TagRFP ( Fig. 4f ). 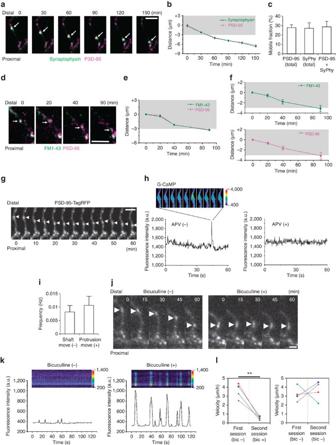Figure 4: Translocation of synaptic contact sites regulated by neuronal activity. (a–c) Coordinated movement of a presynaptic bouton detected by synaptophysin-CFP fluorescence and a postsynaptic PSD-95-YFP punctum (arrows ina). The graph inbindicates the coordinated change in the position of the presynaptic and postsynaptic components. The fraction of mobile pairs of PSD-95-YFP and synaptophysin-CPF (29±6%,n=7 cells) was comparable with the total mobile fraction of PSD-95-YFP (28±3%,n=7 cells) and synaptophysin-CFP (27±6%,n=7 cells) (c). (d–f) Coordinated movement of an FM1-43 punctum and a PSD-95-TagRFP punctum (arrows ind). The graph ineindicates the coordinated change in the position of two fluorescent puncta. The averaged positions of mobile FM1-43 and PSD-95-TagRFP puncta (f) are also highly coordinated with similar velocities (FM1-43: 2.1±0.4 μm h−1; PSD-95: 2.1±0.5 μm h−1;n=4 cells from four culture preparations). (g–i) NMDA receptor-dependent local calcium transients at the sites of mobile PSD-95 puncta. Translocation of PSD-95-TagRFP puncta along the dendritic protusions (arrowheads ing) was monitored simultaneously with local calcium transients detected by G-CaMP6 (h). G-CaMP6 images correspond to the time point of 5 min ing. The frequency of the local calcium transients was comparable between mobile PSD-95 puncta and stationary PSD-95 puncta in dendritic shafts (i; 0.63±0.20 versus 0.48±0.15 min−1,n=11 puncta from four independent experiments for both protrusions and shafts). Application of APV completely suppressed local calcium transients (no event in four experiments). (j–l) Increased spontaneous firing evoked by bicuculline blocked synapse translocation. Translocation of PSD-95-TagRFP was monitored before and after application of bicuculline (arrowheads inj). Bicuculline treatment induced global calcium transients detected by G-CaMP6 (k), possibly corresponding to bursts of action potentials. Comparison of the puncta velocity revealed a reduction in mobility under bicuculline treatment (l;n=4 cells from four independent experiments for both conditions). Significant differences (paired Student'st-test): **P<0.01. Scale bars, 5 μm fora,d,g, 2 μm forj. All numeric data are mean±s.e.m. Figure 4: Translocation of synaptic contact sites regulated by neuronal activity. ( a – c ) Coordinated movement of a presynaptic bouton detected by synaptophysin-CFP fluorescence and a postsynaptic PSD-95-YFP punctum (arrows in a ). The graph in b indicates the coordinated change in the position of the presynaptic and postsynaptic components. The fraction of mobile pairs of PSD-95-YFP and synaptophysin-CPF (29±6%, n =7 cells) was comparable with the total mobile fraction of PSD-95-YFP (28±3%, n =7 cells) and synaptophysin-CFP (27±6%, n =7 cells) ( c ). ( d – f ) Coordinated movement of an FM1-43 punctum and a PSD-95-TagRFP punctum (arrows in d ). The graph in e indicates the coordinated change in the position of two fluorescent puncta. The averaged positions of mobile FM1-43 and PSD-95-TagRFP puncta ( f ) are also highly coordinated with similar velocities (FM1-43: 2.1±0.4 μm h −1 ; PSD-95: 2.1±0.5 μm h −1 ; n =4 cells from four culture preparations). ( g – i ) NMDA receptor-dependent local calcium transients at the sites of mobile PSD-95 puncta. Translocation of PSD-95-TagRFP puncta along the dendritic protusions (arrowheads in g ) was monitored simultaneously with local calcium transients detected by G-CaMP6 ( h ). G-CaMP6 images correspond to the time point of 5 min in g . The frequency of the local calcium transients was comparable between mobile PSD-95 puncta and stationary PSD-95 puncta in dendritic shafts ( i ; 0.63±0.20 versus 0.48±0.15 min −1 , n =11 puncta from four independent experiments for both protrusions and shafts). Application of APV completely suppressed local calcium transients (no event in four experiments). ( j – l ) Increased spontaneous firing evoked by bicuculline blocked synapse translocation. Translocation of PSD-95-TagRFP was monitored before and after application of bicuculline (arrowheads in j ). Bicuculline treatment induced global calcium transients detected by G-CaMP6 ( k ), possibly corresponding to bursts of action potentials. Comparison of the puncta velocity revealed a reduction in mobility under bicuculline treatment ( l ; n =4 cells from four independent experiments for both conditions). Significant differences (paired Student's t -test): ** P <0.01. Scale bars, 5 μm for a , d , g , 2 μm for j . All numeric data are mean±s.e.m. Full size image We next examined the presence of NMDA ( N -methyl- D -aspartate) receptor-dependent local calcium transient at the moving PSD-95 clusters. We expressed a genetically encoded calcium sensor G-CaMP6 in dissociated neurons together with PSD-95-TagRFP and monitored the movement of PSD-95-TagRFP puncta ( Fig. 4g ) together with G-CaMP6 fluorescence ( Fig. 4h ). At the sites of PSD-95 puncta, local calcium transients could be detected in an Mg ++ -free solution containing tetrodotoxin (TTX), and these calcium signals were completely abolished by application of the NMDA receptor antagonist 2-amino-5-phosphonovaleric acid (APV). The frequency of local calcium transients at the translocating PSD-95 puncta was similar to that at the stationary PSD-95 puncta on dendritic shafts ( Fig. 4i ). The presence of surface NMDA receptors within the translocating PSD-95 clusters and that of active presynaptic vesicle recycling as revealed by FM1-43 dye loading indicate translocation of functional pre- and postsynaptic components along the dendritic protrusions. Involvement of dendritic microtubules in retrograde PSD mobility Recent studies indicated stochastic entry of microtubules into filopodia/spines in pyramidal neurons [17] , [18] . Specific long-range movement of PSD-95 puncta along interneuron protrusions may require microtubule-dependent mobility. To test this, we transfected dissociated hippocampal neurons with the microtubule plus-tip protein EB3 tagged with GFP (EB3-GFP) [19] and monitored movement of the plus ends within dendrites. Anterograde movement of EB3-GFP within dendritic protrusions was frequently observed, indicating microtubule growth towards the distal ends of protrusions ( Fig. 5a ). Specific staining of dendritic protrusions with anti-tubulin was not possible because of the overlap with axonal microtubules. Therefore, we performed immunocytochemistry using anti-MAP2 antibody and confirmed the presence of MAP2 in the protrusions containing mobile PSD-95 puncta ( Fig. 5b ). Electron microscopic analysis confirmed the presence of microtubules in dendritic protrusions containing PSD-95-GFP puncta ( Fig. 5c–e ). To confirm the role of microtubules in PSD mobility, time-lapse images of PSD puncta were recorded before and after pharmacological perturbation using either latrunculin A or vincristine, agents known to disrupt actin- and microtubule-dependent transport, respectively ( Fig. 5f ) [20] . The fraction of mobile PSD puncta was smaller in neurons treated with vincristine, whereas latrunculin A tended to increase the relative number of mobile PSD puncta, but the effect was not statistically significant. These results implicate microtubule-dependent transport in the mobility of PSD-95 puncta along dendritic protrusions. 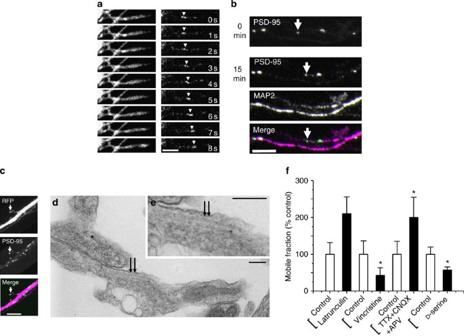Figure 5: Microtubules in dendritic protrusions are involved in PSD mobility. (a) Time-lapse imaging of an EB3-GFP and RFP-expressing neuron showing penetration of an EB3-GFP comet (arrowheads) into a dendritic protrusion. Scale bar, 5 μm. (b) Immunocytochemical staining of interneurons with an anti-MAP2 antibody after time-lapse imaging of PSD-95-GFP. Arrows indicate a PSD-95-GFP punctum moving along a MAP2-positive protrusion. The neuron was fixed 15 min after live imaging. Scale bar, 5 μm. (c–e) Electron micrograph showing microtubules within a dendritic protrusion (double arrows indande) of an interneuron. The neuron expressing PSD-95-GFP and RFP was imaged to confirm the presence of PSD-95 puncta in a dendritic protrusion (arrows inc). The same protrusion was identified under an electron microscope to reveal the detail of the cytoplasmic structure. This dendritic protrusion was apposed to a presynaptic bouton filled with synaptic vesicles (asterisk ind). Scale bars, 5 μm for light microscopic images, 200 nm for electron micrographs. (f) Pharmacological manipulation of retrograde PSD mobility. Perturbation of microtubules by vincristine (1 μM) decreased the mobile fraction of PSD-95 puncta, whereas actin perturbation by latrunculin A (5 μM) tended to enhance PSD mobility. Blockade of both voltage-gated sodium channels and ionotropic glutamate receptors by applying a mixture of TTX (1 μM), CNQX (10 μM) and APV (50 μM) increased the mobile fraction of PSDs. Activation of NMDA-type glutamate receptors byD-serine (10 μM) inhibited PSD mobility. (n=5 cells for all the conditions.) Significant differences (paired Student'st-test): *P<0.05. All numeric data are mean±s.e.m. Figure 5: Microtubules in dendritic protrusions are involved in PSD mobility. ( a ) Time-lapse imaging of an EB3-GFP and RFP-expressing neuron showing penetration of an EB3-GFP comet (arrowheads) into a dendritic protrusion. Scale bar, 5 μm. ( b ) Immunocytochemical staining of interneurons with an anti-MAP2 antibody after time-lapse imaging of PSD-95-GFP. Arrows indicate a PSD-95-GFP punctum moving along a MAP2-positive protrusion. The neuron was fixed 15 min after live imaging. Scale bar, 5 μm. ( c – e ) Electron micrograph showing microtubules within a dendritic protrusion (double arrows in d and e ) of an interneuron. The neuron expressing PSD-95-GFP and RFP was imaged to confirm the presence of PSD-95 puncta in a dendritic protrusion (arrows in c ). The same protrusion was identified under an electron microscope to reveal the detail of the cytoplasmic structure. This dendritic protrusion was apposed to a presynaptic bouton filled with synaptic vesicles (asterisk in d ). Scale bars, 5 μm for light microscopic images, 200 nm for electron micrographs. ( f ) Pharmacological manipulation of retrograde PSD mobility. Perturbation of microtubules by vincristine (1 μM) decreased the mobile fraction of PSD-95 puncta, whereas actin perturbation by latrunculin A (5 μM) tended to enhance PSD mobility. Blockade of both voltage-gated sodium channels and ionotropic glutamate receptors by applying a mixture of TTX (1 μM), CNQX (10 μM) and APV (50 μM) increased the mobile fraction of PSDs. Activation of NMDA-type glutamate receptors by D -serine (10 μM) inhibited PSD mobility. ( n =5 cells for all the conditions.) Significant differences (paired Student's t -test): * P <0.05. All numeric data are mean±s.e.m. Full size image We next tested if neuronal activity is involved in the regulation of PSD mobility. Blockade of both voltage-gated sodium channels and ionotropic glutamate receptors significantly enhanced PSD movement, while activation of NMDA-type glutamate receptors by the co-agonist D -serine suppressed PSD movement ( Fig. 5f ). To induce more physiological activity in the neuronal network, GABAergic transmission was blocked by applying the GABA A receptor antagonist bicuculline. This treatment induced repetitive firing of neurons that could be monitored by G-CaMP6 fluorescence ( Fig. 4k ). PSD-95-TagRFP puncta within dendritic protrusions became significantly less motile after application of bicuculline ( Fig. 4j,l ), indicating that synaptic activity suppresses synaptic translocation. LIS1-dependent retrograde PSD mobility in dissociated neurons Our results in dissociated neurons indicated the presence of growing microtubules with plus ends distal in dendritic protrusions. It is thus likely that PSD translocation is regulated by minus-end-directed motors, such as dynein molecules. Therefore, we evaluated the role of LIS1, a known regulator of the dynein motor complex [15] , [16] . Both LIS1 and its interacting protein NDEL1 are expressed in the postnatal brain and enriched in the purified PSD fraction [21] , [22] . First, we assessed the effect of LIS1 and NDEL1 knockdown using targeted short hairpin RNAs in dissociated hippocampal neurons at 9 DIV. LIS1 and NDEL1 knockdown did not impair the normal development of dendrites, but significantly reduced the fraction of mobile PSD-95-GFP puncta ( Fig. 6a ). Impaired PSD-95 mobility was rescued by overexpression of interfering RNA (RNAi)-insensitive LIS1 and NDEL1 mutants, confirming the specificity of the knockdown. 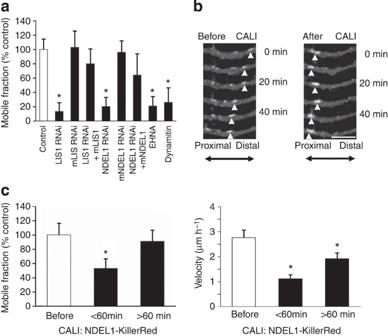Figure 6: Effect of manipulating LIS1/NDEL1/dynein activity in interneurons on PSD mobility. (a) Fraction of mobile PSD puncta in interneurons transfected with PSD-95-GFP and RFP (control) or PSD-95-GFP, RFP and respective short hairpin RNA (shRNA) constructs. Two additional methods for inhibiting dynein-based mobility were also included (treatment with 1 mM erythro-9-[3-(2-hydroxynonyl)] adenine (EHNA) and dynamitin transfection). PSD mobility was suppressed by LIS1 or NDEL1 shRNA and rescued by overexpression of RNAi-insensitive LIS1 and NDEL1 mutants ('LIS1 RNAi+mLIS1' and 'NDEL1 RNAi+mNDEL1'). Mutant LIS1 and NDEL1 RNAi constructs containing three mismatched nucleotides ('mLIS1 RNAi' and 'mNDEL1 RNAi') did not suppress PSD mobility. Both EHNA treatment and expression of dynamitin suppressed PSD mobility. (n=18 cells for control,n=6 cells for LIS1 RNAi,n=7 cells for mLIS1 RNAi,n=6 cells for LIS1 RNAi+mLIS1,n=8 cells for NDEL1 RNAi,n=5 cells for mNDEL1 RNAi,n=5 cells for NDEL1 RNAi+mNDEL1,n=5 cells for EHNA treatment,n=5 cells for dynamitin transfection.) Significant differences (one-way analysis of variance (ANOVA) followed by Tukey–Kramer multiple comparison tests): *P<0.05. (b) Time-lapse imaging of an interneuron expressing PSD-95-GFP with NDEL1-KillerRed before and after CALI (within 60 min after irradiation). Arrowheads indicate the position of a PSD-95-GFP punctum. Scale bar, 5 μm. (c) Suppression of PSD mobility by CALI of NDEL1-KillerRed. The effect of CALI on the mobile fraction was significant at 5–50 min after CALI (53±13.4%,n=6 cells). The fraction of motile PSD-95-GFP puncta returned to the control level at 60–105 min after CALI (91±15.6%,n=6 cells). The mean velocity of mobile PSD puncta also decreased after CALI and this effect was sustained for more than 60 min (2.8±0.30 μm h−1before CALI, 1.1±0.17 μm h−1at 5–50 min after CALI, 1.9±0.24 μm h−1at 60–105 min after CALI,n=6 cells). Significant differences (one-way ANOVA followed by Tukey–Kramer multiple comparison tests): *P<0.05. All numeric data are mean±s.e.m. Figure 6: Effect of manipulating LIS1/NDEL1/dynein activity in interneurons on PSD mobility. ( a ) Fraction of mobile PSD puncta in interneurons transfected with PSD-95-GFP and RFP (control) or PSD-95-GFP, RFP and respective short hairpin RNA (shRNA) constructs. Two additional methods for inhibiting dynein-based mobility were also included (treatment with 1 mM erythro-9-[3-(2-hydroxynonyl)] adenine (EHNA) and dynamitin transfection). PSD mobility was suppressed by LIS1 or NDEL1 shRNA and rescued by overexpression of RNAi-insensitive LIS1 and NDEL1 mutants ('LIS1 RNAi+mLIS1' and 'NDEL1 RNAi+mNDEL1'). Mutant LIS1 and NDEL1 RNAi constructs containing three mismatched nucleotides ('mLIS1 RNAi' and 'mNDEL1 RNAi') did not suppress PSD mobility. Both EHNA treatment and expression of dynamitin suppressed PSD mobility. ( n =18 cells for control, n =6 cells for LIS1 RNAi, n =7 cells for mLIS1 RNAi, n =6 cells for LIS1 RNAi+mLIS1, n =8 cells for NDEL1 RNAi, n =5 cells for mNDEL1 RNAi, n =5 cells for NDEL1 RNAi+mNDEL1, n =5 cells for EHNA treatment, n =5 cells for dynamitin transfection.) Significant differences (one-way analysis of variance (ANOVA) followed by Tukey–Kramer multiple comparison tests): * P <0.05. ( b ) Time-lapse imaging of an interneuron expressing PSD-95-GFP with NDEL1-KillerRed before and after CALI (within 60 min after irradiation). Arrowheads indicate the position of a PSD-95-GFP punctum. Scale bar, 5 μm. ( c ) Suppression of PSD mobility by CALI of NDEL1-KillerRed. The effect of CALI on the mobile fraction was significant at 5–50 min after CALI (53±13.4%, n =6 cells). The fraction of motile PSD-95-GFP puncta returned to the control level at 60–105 min after CALI (91±15.6%, n =6 cells). The mean velocity of mobile PSD puncta also decreased after CALI and this effect was sustained for more than 60 min (2.8±0.30 μm h −1 before CALI, 1.1±0.17 μm h −1 at 5–50 min after CALI, 1.9±0.24 μm h −1 at 60–105 min after CALI, n =6 cells). Significant differences (one-way ANOVA followed by Tukey–Kramer multiple comparison tests): * P <0.05. All numeric data are mean±s.e.m. Full size image To confirm the involvement of dynein-dependent mobility in synaptic translocation, we blocked the activity of the dynein motor complex by applying erythro-9-[3-(2-hydroxynonyl)] adenine, a known inhibitor of the dynein ATPase, or by overexpressing dynamitin, a subunit of the dynactin complex that inhibits dynein-dependent mobility by inducing disassembly of the complex [23] , [24] . Interneurons treated with erythro-9-[3-(2-hydroxynonyl)] adenine or transfected with dynamitin showed impaired synaptic translocation ( Fig. 6a ), further supporting the involvement of dynein in PSD mobility. To suppress dynein-dependent mobility locally, we designed LIS1 and NDEL1 tagged with KillerRed, a fluorescent protein that induces chromophore-assisted light inactivation (CALI). Although LIS1-KillerRed expression was toxic, NDEL1-KillerRed expression did not impair the normal development and mobility of PSD-95-GFP puncta. Dendritic protrusions were irradiated with intense green light for 60 s, and time-lapse images of PSD-95-GFP were recorded before, immediately after and 60 min after CALI ( Fig. 6b ). Light-induced damage of NDEL1 decreased the fraction of mobile puncta and their average velocity ( Fig. 6c ). The fraction of motile PSD-95-GFP puncta returned to the control level 60 min after CALI. The average velocity of PSD-95-GFP puncta also partially recovered 60–120 min after irradiation ( Fig. 6c ), suggesting a slow exchange of functional NDEL1 between dendritic shafts and protrusions. Impaired PSD mobility in slices from LIS1 mutant mice To confirm the involvement of LIS1 in PSD mobility, we used an alternative genetic approach. The function of LIS1 was decreased by Cre-dependent excision of the Lis1 allele in slice cultures. Mutant mice heterozygous for a conditional knockout/hypomorphic allele ( Lis1 hc/+ ) showed normal cortical development. After Cre-dependent excision of a single Lis1 allele, however, the resulting heterozygous mutants ( Lis1 −/+ ) exhibited clear structural disorganization of the cortex [25] . To visualize PSD puncta in Cre-active neurons, expression plasmids for Cre and PSD-95-GFP were introduced into cortical slice preparations by electroporation. The activity of Cre recombinase was confirmed by including an indicator plasmid that expresses RFP only after removal of a loxP-transcription stopper-loxP sequence by Cre recombinase activity ( Supplementary Fig. S3 ). To reveal synapse remodelling in Lis1 −/+ interneurons, we performed time-lapse imaging experiments at 4–9 DIV. The overall density and dynamics of dendritic protrusions were indistinguishable between Lis1 −/+ and wild-type neurons (density: 0.17±0.015 per μm in wild type and 0.19±0.030 per μm in Lis1 −/+ , lifetime: 19.6±3.9 min in wild type and 21.1±5.6 min in Lis1 −/+ ; n =12 cells for wild type and n =9 cells for Lis1 −/+ ). However, the fraction of PSD puncta localized in the protrusions was reduced in Lis1 −/+ neurons (18.8±3.5% in wild type and 6.7±2.4% in Lis1 −/+ , n =12 and 9 cells). Furthermore, when PSD puncta were present within protrusions, their mobility was significantly suppressed ( Fig. 7a,b ). 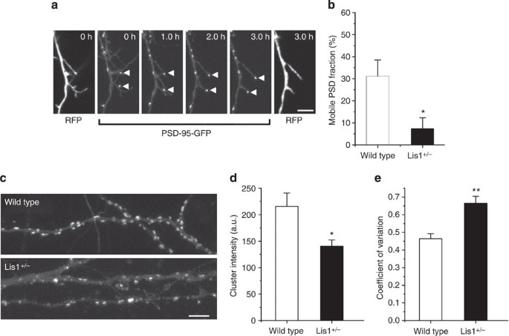Figure 7: Effect of manipulating theLis1gene in cortical slices. (a) Time-lapse images of an interneuron maintained in cortical slices from aLis1hc/+mouse and transfected with expression plasmids encoding Cre recombinase and PSD-95-GFP, together with a Cre indicator plasmid. Arrowheads indicate stationary PSD puncta within dendritic protrusions. Scale bar, 5 μm. (b) Fraction of mobile PSD-95-GFP puncta in dendritic protrusions of control andLis1−/+interneurons (31.2±7.3% for wild type and 7.4±4.9% forLis1−/+,n=12 cells in nine slice cultures for wild type,n=9 cells in nine slice cultures forLis1−/+). Significant differences (unpaired Student'st-test): *P<0.05. (c) Distribution and morphology of PSD-95-GFP puncta in cortical interneurons from wild-type orLis1hc/+mice and transfected with expression plasmids encoding Cre recombinase and PSD-95-GFP, together with a Cre indicator plasmid. Scale bar, 5 μm. (d) Total fluorescence of individual PSD-95-GFP puncta was lower in interneurons of theLis1−/+genotype than in wild-type interneurons (Lis1−/+: 140±12 a.u.,n=28 cells in seven slice cultures; wild type: 215±25 a.u.,n=27 cells from seven slice cultures). Significant differences (unpaired Student'st-test): *P<0.05. (e) Larger variation in the total fluorescence of PSD-95 puncta in interneurons carrying theLis1−/+genotype. The average coefficient of variation for the total fluorescence of PSD-95 puncta in each dendrite was significantly larger inLis1−/+interneurons (Lis1−/+: 0.66±0.039,n=27 cells from seven slice cultures; wild type: 0.46±0.029,n=28 cells from seven slice cultures). Significant differences (unpaired Student'st-test): **P<0.01. All numeric data are mean±s.e.m. Figure 7: Effect of manipulating the Lis1 gene in cortical slices. ( a ) Time-lapse images of an interneuron maintained in cortical slices from a Lis1 hc/+ mouse and transfected with expression plasmids encoding Cre recombinase and PSD-95-GFP, together with a Cre indicator plasmid. Arrowheads indicate stationary PSD puncta within dendritic protrusions. Scale bar, 5 μm. ( b ) Fraction of mobile PSD-95-GFP puncta in dendritic protrusions of control and Lis1 −/+ interneurons (31.2±7.3% for wild type and 7.4±4.9% for Lis1 −/+ , n =12 cells in nine slice cultures for wild type, n =9 cells in nine slice cultures for Lis1 −/+ ). Significant differences (unpaired Student's t -test): * P <0.05. ( c ) Distribution and morphology of PSD-95-GFP puncta in cortical interneurons from wild-type or Lis1 hc/+ mice and transfected with expression plasmids encoding Cre recombinase and PSD-95-GFP, together with a Cre indicator plasmid. Scale bar, 5 μm. ( d ) Total fluorescence of individual PSD-95-GFP puncta was lower in interneurons of the Lis1 −/+ genotype than in wild-type interneurons ( Lis1 −/+ : 140±12 a.u., n =28 cells in seven slice cultures; wild type: 215±25 a.u., n =27 cells from seven slice cultures). Significant differences (unpaired Student's t -test): * P <0.05. ( e ) Larger variation in the total fluorescence of PSD-95 puncta in interneurons carrying the Lis1 −/+ genotype. The average coefficient of variation for the total fluorescence of PSD-95 puncta in each dendrite was significantly larger in Lis1 −/+ interneurons ( Lis1 −/+ : 0.66±0.039, n =27 cells from seven slice cultures; wild type: 0.46±0.029, n =28 cells from seven slice cultures). Significant differences (unpaired Student's t -test): ** P <0.01. All numeric data are mean±s.e.m. Full size image Suppression of PSD mobility in developing dendrites may lead to disorganization of synaptic input patterns in later developmental stages. To test this possibility, we maintained slices prepared from wild-type or mutant mice for 14 days in culture and analysed the distributions of PSD-95-GFP puncta in Cre-active interneurons. Although there were no obvious defects in overall development of dendrites, the distribution of PSD puncta was disorganized in Lis1 −/+ interneurons ( Fig. 7c ). To quantify the genotype-dependent difference, we measured the integrated fluorescence intensity of individual puncta and calculated the mean and coefficient of variation within each dendrite. We found that the mean fluorescence intensity of PSD puncta was reduced, whereas coefficient of variation within each dendrite was higher in interneurons from Lis1 −/+ mice ( Fig. 7d,e ). Thus, the effects of both RNAi-dependent reduction of LIS1 expression and Cre-dependent elimination of a single Lis1 allele confirm that full LIS1 function is essential for PSD mobility and the proper arrangement of PSD puncta in interneuron dendrites. The specific function of a given neural circuit depends on the precise pattern of excitatory, inhibitory and neuromodulatory inputs on neuronal dendrites. The experiments presented in this study revealed that GABAergic interneurons use a microtubule-dependent strategy for synaptic development and organization of excitatory inputs. Immature interneuron dendrites generate protrusions as a means of searching the surrounding tissue microenvironment for appropriate axonal contacts ( Fig. 8b ). After establishing nascent synaptic contacts, these protrusions serve as conduits for the retrograde synapse movement to the parental dendritic shafts ( Fig. 8c ). Tight interaction of presynaptic and postsynaptic plasma membranes may transduce the tension generated in the dendritic protrusions to the presynaptic structure [26] . After reaching the parental dendritic shafts, synapse translocation is downregulated ( Fig. 8d ). Mixed polarity of microtubules in the parental dendritic shafts [27] may suppress directional mobility of synapses. PSD maturation enhances NMDA receptor-dependent calcium influx [28] , which may also negatively regulates PSD mobility. We also provided evidences indicating that precise regulation of dynein function by LIS1 and NDEL1 (ref. 21 ) is critical for regulating synaptic mobility. 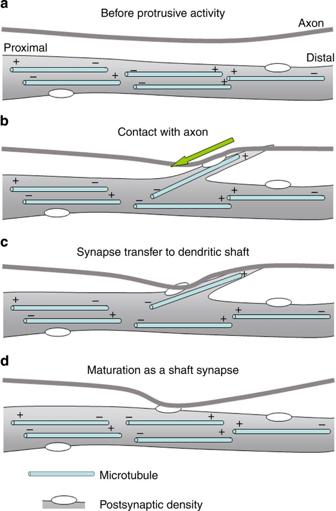Figure 8: Model for coordinated remodelling of dendritic protrusions and PSDs in interneuron dendrites. (a) An interneuron dendrite without protrusions. There is no physical contact with nearby axons. (b) A dendritic protrusion starts contact with a presynaptic axon. Assembly of plus end-distal microtubules in newly formed dendritic protrusions initiate retrograde translocation of PSDs towards the dendritic shafts, while keeping contact with apposed presynaptic boutons. Tight interaction of presynaptic and postsynaptic plasma membranes may transduce the tension generated in the dendritic protrusions to the presynaptic structure. Initiation of PSD mobility may require direct synaptic contacts or diffusible factors released from the axon. (c) Movement of PSDs along dendritic protrusions results in transfer of synapses to the dendritic shaft. (d) On the parental dendritic shafts, where microtubule polarity is mixed, PSD mobility is suppressed and PSD positions are stabilized. It is also possible that activity of the nearby shaft synapses and depolarization of the dendritic shafts contributes to the suppression of PSD mobility. Figure 8: Model for coordinated remodelling of dendritic protrusions and PSDs in interneuron dendrites. ( a ) An interneuron dendrite without protrusions. There is no physical contact with nearby axons. ( b ) A dendritic protrusion starts contact with a presynaptic axon. Assembly of plus end-distal microtubules in newly formed dendritic protrusions initiate retrograde translocation of PSDs towards the dendritic shafts, while keeping contact with apposed presynaptic boutons. Tight interaction of presynaptic and postsynaptic plasma membranes may transduce the tension generated in the dendritic protrusions to the presynaptic structure. Initiation of PSD mobility may require direct synaptic contacts or diffusible factors released from the axon. ( c ) Movement of PSDs along dendritic protrusions results in transfer of synapses to the dendritic shaft. ( d ) On the parental dendritic shafts, where microtubule polarity is mixed, PSD mobility is suppressed and PSD positions are stabilized. It is also possible that activity of the nearby shaft synapses and depolarization of the dendritic shafts contributes to the suppression of PSD mobility. Full size image Various neuronal types in the brain develop dendrites without spines, but it is not clear whether transfer of synapses to dendritic shafts via specialized protrusions is a common mechanism. The aspiny dendrites of tectal neurons in zebrafish show a distinct pattern of PSD formation and dendrite development, [29] in which new PSD puncta are formed exclusively on dendritic filopodia. Subsequent transformation of filopodia into dendritic branches is the major mechanism for synaptic development. The complex dendritic arbourization of zebrafish tectal neurons may be sufficient to maximize connectivity with surrounding axons. In contrast, the dendrites of mammalian cortical interneurons develop fewer branches, and their ability to search surrounding axons and form synapses would likely be limited if they did not extend long protrusions and then transfer the synaptic contacts to the dendritic shafts. A more fundamental question is how dendritic protrusive activity and synapse maturation are controlled in specific neuronal types [30] . The filopodia on pyramidal neurons may also function as conduits for retrograde synapse translocation, as indicated by imaging studies of retrograde PSD movement along such dendritic protrusions [31] , [32] , [33] . Electron microscopic studies of pyramidal neurons in vivo proposed the transfer of synapses formed onto filopodia-like protrusions to dendritic shafts [7] , [9] . The different outcomes of synapse transfer between two neuron types may reflect the affinity of PSDs with cytoskeletal components. For example, pyramidal neuron PSDs may have a higher affinity for actin filaments, which could promote the formation of dendritic spines at the vicinity of PSDs after their transfer to the shafts. We present several lines of evidence indicating that the dynamic behaviour of PSD puncta in interneuron dendrites is distinct from the mobility of non-synaptic scaffold complexes before their recruitment to synaptic contact sites. First, we observed the velocity of PSD puncta to be 2–5 μm h −1 , much slower than the reported velocity of non-synaptic scaffold complexes [34] . Second, the direction of PSD translocation in interneurons was always towards the proximal ends of dendritic protrusions. In contrast, non-synaptic scaffold complexes reportedly move bidirectionally [34] . Third, 78–91% of PSD puncta in interneuron dendritic protrusions also stained positively for presynaptic markers, indicating that most of the imaged PSD puncta were part of synaptic structures. Finally, our time-lapse imaging of presynaptic and postsynaptic structures using PSD-95-YFP and synaptophysin-CFP clearly demonstrated their coordinated movement. Collectively, these findings indicate that the motile behaviour of synaptic junctions on interneuron dendritic protrusions is distinct from the previously reported mobility of non-synaptic scaffold complexes. The movement of PSDs along dendritic protrusions (2–5 μm h −1 ) is slower than dynein-driven fast organelle transport [35] , but comparable to slow high-load transport, such as nucleokinesis and centrosomal movement (5–10 μm h −1 ) [36] . Both LIS1 and NDEL1 are known to be involved in dynein-dependent slow transport of intracellular structures [21] , [22] , [37] , but their roles in rapid organelle transport have been reported to be minimal [38] , [39] or indirect [40] . LIS1 dysfunction leads to impairment of cell migration and nucleokinesis [15] , [16] , reorientation of the entire microtubule system during mitosis [41] , and aberrant centrosome and kinetochore dynamics [42] , [43] . These previous data are consistent with the idea that the PSD translocation we reported here belongs to slow high-load transport and depends on LIS1 and NDEL1. LIS1 and NDEL1 may help dynein-dependent tethering of microtubules at the PSDs. Alternatively, LIS1 and NDEL1 may increase total force of multiple dynein molecules associated with PSDs [21] , [44] . This mechanism may be required to overcome large mechanical resistance generated by interaction of PSDs with both presynaptic components and the surrounding cortical actin meshwork. Indeed, actin depolymerization using latrunculin A tended to enhance PSD movement along dendritic protrusions. Overall, our results indicate the essential role of postsynaptic dynein–NDEL1–LIS1 complex in slow high-load retrograde translocation of the entire synaptic junctions. Our observations indicate that regulation of dynein function by the coordinated activity of LIS1 and NDEL1 (ref. 45 ) is critical for determining the synaptic distribution on interneuron dendrites. Dysfunction of glutamatergic synapses on interneurons may lead to pathogenic disruption of the balance between excitatory and inhibitory synaptic transmission [46] . Indeed, epilepsy is common in human type 1 lissencephaly, a genetic disorder caused by heterozygous loss or mutation of the Lis1 gene [47] . We speculate that defects in LIS1-dependent regulation of synaptic mobility may promote epilepsy by disrupting excitatory inputs onto GABAergic interneurons in addition to the known effects of LIS-1 loss-of-function on the migration of early postmitotic neurons. This new aspect of LIS1 function may be important to our understanding of the pathophysiology of lissencephaly and help define new therapeutic targets. Cultures. Cultures of dissociated hippocampal neurons from 17-day-old embryonic mice were prepared as described previously [48] . Mouse cortical slice cultures were prepared from 0- to 2-day-old wild-type mice, GAD67-GFP knockin mice [49] and Lis1 hc/+ mice [25] as described previously [50] . In brief, dissected brains were cut into 300-μm slices using a tissue slicer, placed on transparent porous filters (Ominipore filters, Millipore, Bedford, MA, USA) in a 5% CO 2 humid incubator at 34 °C and fed every third day with culture medium containing 48% Eagle's basal medium, 24% Earle's balanced salt solution and 24% horse serum supplemented with 5 mg ml −1 glucose, 10 mM HEPES, 1 mM L -glutamine, 50 U ml −1 penicillin and 50 U ml −1 streptomycin. Molecular constructs and gene expression. Constructs of PSD-95-GFP, PSD-95-YFP, synaptophysin-CFP and GFP-Homer1c were described previously [6] , [48] , [51] . EB3 and NDEL1 were amplified by PCR and the sequences were verified by DNA sequencing. PSD-95-TagRFP, PSD-95-Dronpa, EB3-GFP and NDEL1-KillerRed were generated by inserting the full coding region into the TagRFP, Dronpa-Green, pEGFP or KillerRed vector (Evrogen JSC, Moscow, Russia; MBL, Nagoya, Japan; Clontech, Mountain View, CA, USA). For neuronal expression of GFP-tagged proteins, the DNA fragments containing coding regions of GFP-tagged proteins were inserted into the multiple cloning site of a vector with the upstream β-actin promoter sequences [52] . G-CaMP6 is a modified version of genetically encoded calcium sensor G-CaMP [53] with increased dynamic range (M. O, T. Sasaki, J.Sadakari, K.Ando, Y. Kagawa-Nagamura, Y. Ikegaya & J.N unpublished results). Transfection of hippocampal neurons was performed using Effectene transfection reagent (Qiagen, Hilden, Germany) or the calcium phosphate method 4 days after plating [54] . Recombinant adenoviruses for expression of PSD-95-YFP and synaptophysin-CFP were described previously [6] . Transfection of expression plasmids encoding PSD-95-GFP, GFP-Homer1c or RFP into slices was performed as described previously [55] . RNA interference. Small interfering RNA (siRNA) sequences targeting LIS1 and NDEL1 were described previously [56] . The oligonucleotides were subcloned into the pSilencer siRNA expression vector (Ambion, Austin, TX, USA) to generate short hairpin RNA constructs and transfected into primary hippocampal neurons using Effectene transfection reagent on day 4 after plating [54] . Immunocytochemistry and electron microscopy. Dissociated cells were fixed in 2% paraformaldehyde in PBS for 25 min, permeabilized with 0.2%. Triton X-100 for 5 min, blocked with 5% normal goat serum and incubated with monoclonal anti-GAD67 (Chemicon, Temecula, CA, USA), monoclonal anti-MAP2 (Sigma, St Louis, MO, USA), polyclonal anti-synapsin I (Chemicon), polyclonal anti-synaptophysin (Zymed Laboratories, San Francisco, CA, USA), polyclonal anti-vGLUT1 or monoclonal anti-bassoon (Stressgen Bioreagents, Brussels, Belgium) for 60 min. Slices were fixed in 2% paraformaldehyde in PBS for 60 min, permeabilized and blocked with 1.0% Triton X-100 plus 5% normal goat serum in PBS for 60 min, and incubated with anti-synapsin I or anti-synaptophysin overnight at 4 °C The primary antibody was visualized using Alexa 546 or Alexa633-conjugated goat anti-mouse IgG or anti-rabbit IgG (Invitrogen, Carlsbad, CA, USA). For electron microscopy, hippocampal cultures were fixed for 1 h in 0.1 M PBS containing 1.0% glutaraldehyde and 4% paraformaldehyde for 1 h. Post fixation with 1.0% OsO 4 , dehydration and embedding in epoxy resin, 60- to 80-nm-thick sections were prepared and examined. Imaging of dissociated hippocampal neurons. Live cells were mounted in a chamber at 37 °C with a continuous flow of humidified 5% CO 2 to maintain the pH of the medium during prolonged time-lapse experiments. Imaging of neurons in saline solutions containing HEPES buffer were performed in the same chamber without 5% CO 2 aeration. Images were obtained using a Fluoview confocal laser-scanning microscope (Olympus, Tokyo, Japan) with ×60 or ×100 oil immersion lenses. FM1-43 loading was performed by exposing neurons to the dye (15 μM) in high K + solution (75 mM NaCl, 70 mM KCl, 2 mM CaCl 2 , 2 mM MgCl 2 , 5 mM HEPES and 20 mM glucose (pH 7.4)) for 2 min and then switching to a normal saline solution (140 mM NaCl, 5 mM KCl, 2 mM CaCl 2 , 2 mM MgCl 2 , 5 mM HEPES and 20 mM glucose (pH 7.4)) containing 1 μM TTX. Imaging of local calcium transients was performed by perfusing neurons with a Mg 2+ -free solution (140 mM NaCl, 5 mM KCl, 4 mM CaCl 2 , 0 mM MgCl 2 , 5 mM HEPES and 20 mM glucose (pH 7.4)) containing 1 μM TTX. NMDA receptor-dependent calcium influx was blocked with 100 μM APV. To induce spontaneous firing, cells were perfused with a normal saline solution containing 20 μM bicuculline. To initiate CALI of NDEL1, a small segment of dendrites was illuminated with green light (515–560 nm) from a mercury lamp. This procedure did not affect the number of newly generated dendritic protrusions per hour and lifetime of protrusions in interneurons expressing both NDEL1-KillerRed and PSD-95-GFP. Imaging of slice culture preparations. Live hippocampal slice cultures were mounted in a microscope stage chamber containing low-serum medium (MEM supplemented with 5% FCS, 10 mM HEPES, 50 U ml −1 penicillin and 50 U ml −1 streptomycin). The temperature of the medium was maintained at 34 °C, and the stage chamber was aerated with 5% humidified CO 2 . Simultaneous imaging of GFP-tagged PSD proteins and RFP was performed using the Fluoview confocal laser-scanning microscope with a ×60 water-immersion lens (NA, 1.0). Fluorophores were excited using the 488-nm line of an argon laser and the 543-nm line of a HeNe laser. Image analysis. Image processing and analysis was performed using Metamorph software (Molecular Devices, Sunnyvale, CA, USA). For analysis of the morphology and dynamics of dendritic protrusions, single-channel RFP image stacks, acquired at 3-min or 10-min intervals, were selected. Image stacks consisting of 8–12 images with different focal planes were projected into a single image using a maximum brightness operation. These projected images were aligned manually to correct for drift in the XY plane. Lengths of all protrusions in the projected images were determined by tracing the protrusions manually. Lifetimes were defined as the number of frames in which a particular protrusion was visible and expressed in minutes. PSD-95-GFP and GFP-Homer1c puncta were identified in the projection images as local increases in fluorescence intensity >0.2 μm 2 . The XY coordinates of each fluorescent punctum were recorded from consecutive time-lapse images, and the distance and average velocity of movement was calculated. Puncta showing unidirectional movement >3 μm within 2 h towards the parental dendritic shafts were classified as mobile puncta. For analysis of translocation of PSD-95-YFP puncta together with synaptophysin-CFP puncta, we identified fluorescent puncta in two channels independently and judged apposition by pixel overlap. To reduce selection bias, extraction of fluorescent puncta was performed automatically using Metamorph software with an identical setting of thresholding. The dendritic protrusions were manually identified and measured by multiple investigators blind to genotypes, culture conditions and GAD67-GFP expression. When equal numbers of dendritic protrusions/puncta were selected for further analyses, random selection was performed. Statistical analysis. Data are presented as means±standard error. Paired means were compared using t -tests. Multiple means were compared using analysis of variance followed by Tukey–Kramer post hoc multiple comparison tests. How to cite this article: Kawabata, I. et al . LIS1-dependent retrograde translocation of excitatory synapses in developing interneuron dendrites. Nat. Commun. 3:722 doi: 10.1038/ncomms1736 (2012).